Sophisticated digestive systems in early arthropods Understanding the way in which animals diversified and radiated during their early evolutionary history remains one of the most captivating of scientific challenges. Integral to this is the ‘Cambrian explosion’, which records the rapid emergence of most animal phyla, and for which the triggering and accelerating factors, whether environmental or biological, are still unclear. Here we describe exceptionally well-preserved complex digestive organs in early arthropods from the early Cambrian of China and Greenland with functional similarities to certain modern crustaceans and trace these structures through the early evolutionary lineage of fossil arthropods. These digestive structures are assumed to have allowed for more efficient digestion and metabolism, promoting carnivory and macrophagy in early arthropods via predation or scavenging. This key innovation may have been of critical importance in the radiation and ecological success of Arthropoda, which has been the most diverse and abundant invertebrate phylum since the Cambrian. Ecdysozoans (moulting animals) including priapulid worms, lobopodians and arthropods have been ubiquitous in marine communities since the Cambrian and are the most successful clade of present-day animals, inhabiting aquatic, terrestrial and aerial ecological niches [1] . Their remarkable and rapid success raises the question of identifying which triggers and factors shaped their early evolutionary history. Studies based on genomic data [1] , [2] , [3] and fossil evidence from Cambrian exceptional biota [4] , [5] , [6] , [7] , [8] , [9] , [10] suggest a sister-group relationship between arthropods and onychophorans (and possibly tardigrades), with at least some lobopodians occupying basal positions in an arthropod stem lineage of Cambrian fossil taxa that depicts the gradual acquisition of arthropod features. Palaeontological evidence has mainly focused on the evolution of external features, such as cephalization [8] , [9] , arthrodization [6] and arthropodization [4] , [5] , and discussed the degree to which these served as critical steps in the radiation of arthropods. The recent discovery of brains and nervous systems preserved in Cambrian arthropods demonstrates that internal anatomical systems also provide valuable information for understanding character evolution and the timing of otherwise elusive key innovations [11] , [12] . Here we collate records of exceptionally preserved, complex digestive organs in new and previously described specimens of early stem group arthropods from the Early Cambrian Chengjiang ( Megadictyon and Jianshanopodia, China [13] ) and Sirius Passet ( Pambdelurion , Greenland [10] , [14] ) biotas that have clear functional similarities to structures in modern crustaceans and in a variety of arthropod lineages from the Cambrian. Reniform structures (RS) acting as gut glands would have increased efficency of food processing, allowing early arthropods to more easily digest large food particles (macrophagy) and maintain the higher energy demands of an active and mobile predatory lifestyle. This innovation may have contributed to the evolutionary success of the arthropods by allowing them to exploit more food resources and modes of life. Our study on digestive systems also emphasizes the importance of internal driving factors in the early steps of animal biodiversification. Large lobopodians with paired reniform structures Megadictyon and Jianshanopodia [15] , [16] , [17] , [18] , [19] , [20] ( Fig. 1 , Supplementary Note 1 and Supplementary Fig. 1 ) from the Chengjiang biota in China are relatively large (length >20 cm) animals that recall modern onychophorans [21] in being superficially annulated and bearing pairs of thick unsegmented lobopods. They have a pair of robust, possibly prehensile frontal appendages armed with a terminal claw and pointed outgrowths along their inner margins ( Supplementary Fig. 2a–e ). Pambdelurion [10] is one of the largest and most common animals (length 40 cm) from the Sirius Passet biota of Greenland and co-occurs with Kerygmachela [22] ( Supplementary Fig. 3 ) of comparable morphology. They differ from Megadictyon and Jianshanopodia in having paired dorsolateral flap-like lobes in addition to corresponding pairs of smaller multi-annulated ventral lobopods ( Fig. 2 , Supplementary Figs 2f–h and 3 ). 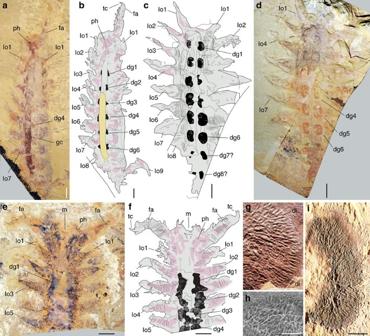Figure 1: Digestive glands in Early Cambrian lobopodians from the Chengjiang biota. (a,b)Megadictyoncf.haikouensis, ELI-M001A, with preserved gut contents. (c,d) Undetermined lobopodian, ELI-JS0003, anterior and posterior ends missing. (e,f) Undet. lobopodian, ELI-JS0001, posterior part missing. (g)Jianshanopodia decora,ELI-J0006, details of diverticula network. (h,i) Reniform shape and diverticula in ELI-M002A.his a scanning electron micrograph. Body in grey, presumed muscle remains in pink, digestive glands in black and gut contents in yellow. dg1–8, digestive glands 1–8; fa, frontal appendage; gc, gut content; lo1-9; lobopod 1–9; m, mouth; ph, pharynx; tc, terminal claw. Scale bar, 10 mm fora–f; 1 mm forg,i; and 500 μm forh. New and previously described specimens ( Supplementary Table 1 ) of Megadictyon , Jianshanopodia and Pambdelurion show that these taxa have a cylindrical gut tract flanked with RS composed of a three-dimensional (3D)-preserved network of anastomosing blind diverticula ( Figs 1 and 2 , Supplementary Figs 1 and 4 ). In Megadictyon and Jianshanopodia , these RS are coloured red or black owing to local enrichment in carbon and diagenetic iron oxides, whereas they are composed of calcium phosphate in Pambdelurion (confirmed by scanning electron microscopic energy dispersive spectrometry (SEM-EDS), Supplementary Fig. 5 ). The diverticula form radiating bunches that open into the gut lumen via a primary duct. The diameter of distal diverticula observed in section ( Pambdelurion ) is about 500 μm ( Supplementary Fig. 4h–k ). Eight or nine pairs of RS are distributed evenly along the gut of the Chinese forms, each pair being inserted halfway between the main axis of two successive lobopods, the anteriormost of which lies between the second and third pair of lobopods. They are absent beyond the fourth last lobopod pair. Pambdelurion and Kerygmachela have six and eight pairs of RS, respectively ( Fig. 2 , Supplementary Figs 3 and 4 ). One specimen of Megadictyon has 3D-preserved gut contents, which fill a ~7-cm long section posteriorly, the gut wall delineating a sharp boundary between the gut contents and other body features ( Supplementary Fig. 6 ). Four pairs of RS occur along this particular section. These gut contents are red owing to Fe and C enrichment, and contain numerous platy, often radiating narrow cavities with no preferential orientation ( Supplementary Fig. 6d–j ) and filled with haematite donut-shaped microcrystals (SEM-EDS; Supplementary Fig. 6k–o ). Gut content preservation probably results from the weathering of preexisting minerals, possibly pyrite, that precipitated from organic-rich gut contents in the presence of sulphate-reducing bacteria. Only one specimen of Pambdelurion shows possible undigested exoskeletal fragments of arthropods in its posterior gut ( Supplementary Fig. 4l ). Figure 1: Digestive glands in Early Cambrian lobopodians from the Chengjiang biota. ( a , b ) Megadictyon cf. haikouensis , ELI-M001A, with preserved gut contents. ( c , d ) Undetermined lobopodian, ELI-JS0003, anterior and posterior ends missing. ( e , f ) Undet. lobopodian, ELI-JS0001, posterior part missing. ( g ) Jianshanopodia decora, ELI-J0006, details of diverticula network. ( h , i ) Reniform shape and diverticula in ELI-M002A. h is a scanning electron micrograph. Body in grey, presumed muscle remains in pink, digestive glands in black and gut contents in yellow. dg1–8, digestive glands 1–8; fa, frontal appendage; gc, gut content; lo1-9; lobopod 1–9; m, mouth; ph, pharynx; tc, terminal claw. Scale bar, 10 mm for a – f ; 1 mm for g , i ; and 500 μm for h . 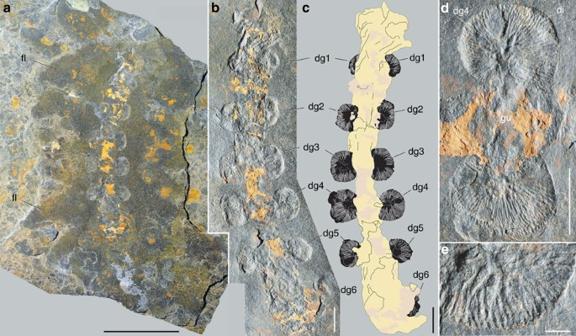Figure 2: Digestive glands in the Early Cambrian lobopodianPambdelurion whittingtonifrom the Early Cambrian Sirius Passet biota. (a–e) MGUH 24514, incomplete specimen with paired digestive glands. (a) General view. (b,c) Close-up of digestive system. (d) Details of the fourth pair of digestive glands. (e) Close-up showing anastomosed diverticula. Gut in pale yellow, presumed muscle remain in pink and digestive glands in black. di, diverticula; dg1–6, digestive glands 1–6; fl, flap-like lobes; gu, gut. Scale bar, 50 mm fora; 10 mm forb,c; 5 mm ford; and 2 mm fore. Full size image Figure 2: Digestive glands in the Early Cambrian lobopodian Pambdelurion whittingtoni from the Early Cambrian Sirius Passet biota. ( a – e ) MGUH 24514, incomplete specimen with paired digestive glands. ( a ) General view. ( b , c ) Close-up of digestive system. ( d ) Details of the fourth pair of digestive glands. ( e ) Close-up showing anastomosed diverticula. Gut in pale yellow, presumed muscle remain in pink and digestive glands in black. di, diverticula; dg1–6, digestive glands 1–6; fl, flap-like lobes; gu, gut. Scale bar, 50 mm for a ; 10 mm for b , c ; 5 mm for d ; and 2 mm for e . Full size image Reniform structures are digestive glands Numerous lobopodian species have paired dorsal or dorsolateral sclerites such as the elongated spines of Hallucigenia [23] , [24] and the ovoid ornamented plates of Microdictyon [25] . Their symmetrical distribution on both sides of the longitudinal axis of the animal recalls that of RS in Jianshanopodia, Megadictyon and Pambdelurion . However, these metameric sclerites were primarily sclerotized or biomineralized [24] , possess a consistent shape with sharp outlines and are found in consistent locations with each pair lying directly above a pair of lobopods. In contrast, RS have irregular outlines and are positioned between successive lobopods. Their radiating network is clearly connected to the gut via primary ducts ( Fig. 2d , Supplementary Fig. 1d ) whereas sclerites are cuticular structures with no relation to internal organs. RS are also unlikely to represent muscles associated with lobopods or their insertion sites. They lack the typical fibrous structure of muscles and do not laterally extend into the lobopods or any other part of the body. Moreover, in Cambrian arthropods where remains of muscles associated with appendages have been described [26] , [27] , these muscles are located abaxial to the digestive glands, which lie closer to the intestinal tract. Muscle scars visible in trilobites [28] with strongly mineralized exoskeletons do not show 3D-radiating patterns comparable to that of RS [29] and are located abaxial to the RS [30] . The Cambrian stem lineage arthropod Anomalocaris also preserves patches of musculature that consist of densely arranged parallel fibres located abaxial to the digestive glands and associated with paired body flaps [26] . Moreover, RS are found only in the central region of the body in both Anomalocaris and the lobopodians, such as in Jianshanopodia where RS are absent anterior to the second pair of lobopods and posterior to the 10th pair of lobopods. The preservation, morphology and connectivity to the intestinal tract suggest that RS are digestive glands. Possible recent functional analogues Comparisons with recent crustaceans also suggest that the RS can be interpreted as midgut glands. Branchiuran crustaceans such as Argulus [31] , [32] possess a large symmetrical network of diverticula that branches off from the anterior midgut, expands laterally into the carapace and closely resembles RS ( Figs 2d and 3a ). The size of each bunch of diverticula is comparable with that of RS in Pambdelurion . The main functions of this structure in branchiurans are food storage (for example, fish blood in the ectoparasite Argulus ), enzymatic breakdown of food via phosphatases, esterases, carbohydrases and proteases, and eventual absorption of nutrients. R-cells and F-cells indicate digestive processes comparable with those occurring in the hepatopancreas of decapods [33] ( Fig. 3g ). The RS are strikingly similar to the extensive arborescent network of diverticula ( Fig. 3b–f ) of phyllosoma larval stages of recent spiny lobsters [34] , within which fluid food is digested via R-cells, and the lateral masses of multibranched midgut diverticula of recent horseshoe crabs [35] , [36] . Although branchiurans and spiny lobsters are highly derived crustaceans with no close phylogenetic relationship to early arthropod fossils, their digestive glands are the closest modern analogues to RS in terms of both morphology and possible function. Accordingly, we interpret RS as serial digestive glands that may have functioned in a similar way as their modern counterparts in crustaceans, with fluidized food entering the diverticula network to be digested by enzymes and assimilated via surrounding tissues. Food entry may have been regulated by peristaltic contractions within the glandular structures, by sphincters near the gut junction or even by pressure exerted from nearby lobopods. The homonomous series of digestive glands in Megadictyon , Jianshanopodia and Pambdelurion has no exact equivalent in modern arthropods. Many arachnids possess comparable numbers of digestive glands, but these structures vary greatly in morphology even within a single individual [37] , [38] . Crustaceans rarely have more than a single pair of digestive glands, which can be extremely developed and occupy much of the trunk (for example, the hepatopancreas of decapods [33] ). Notable exceptions are the remipede crustaceans, as exemplified by Speleonectes [39] , [40] , [41] , which has up to 32 pairs of identical diverticula along its gut. However, these diverticula are simple metameric protrusions of the midgut with no complex structural (for example, tubular network) or histological differentiation [41] . Each pair of diverticula ( Fig. 3h,i ) is inserted in the anterior part of the trunk segment but not in line with the axis of appendages. This recalls the arrangement of digestive glands in the Cambrian lobopodians. 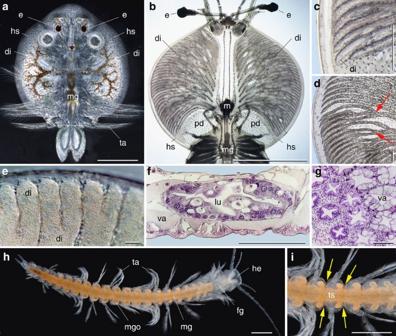Figure 3: Digestive glands in Recent crustaceans. (a)Argulus japonicus(branchiuran ectoparasite) in transmitted light showing paired diverticula filled with fish blood. (b–f) Phyllosoma larval stage of palinurid decapod crustaceans. (b) General view showing symmetrical network of diverticula branching off from midgut. (c) Blind-ended diverticula. (d) Bifurcating diverticula (red arrows). (e) Diverticula filled with fluid food. (f) Histological section through diverticulum (note large vacuoles in digestive cells). (g) Section through the hepatopancreas ofNephrops norvegicus(Decapoda) showing typical closely packed digestive tubules. (h,i)Speleonectesatlantida40(remiped crustacean) from submarine cave, Canary Islands, showing orange-coloured midgut with numerous lateral pairs of outpocketings (yellow arrows indicate segment boundaries). di, diverticula; e, eye; fg, foregut; he, head; hs, head shield; lu, lumen; m, mouth; mg, midgut; mgo, midgut outpocketing; pd, primary duct; ta, trunk appendage; ts, trunk segment; va, vacuole. All light micrographs.a, courtesy A. Avenant-Oldewage;e,f, S. Mikami;g, D.M. Neil;h,i, U. Streker,http://www.naturalanza.com. Scale bar, 5 mm forb,h,i; 1 mm fora,c; 500 μm ford, 100 μm fore,f; and 25 μm forg. Figure 3: Digestive glands in Recent crustaceans. ( a ) Argulus japonicus (branchiuran ectoparasite) in transmitted light showing paired diverticula filled with fish blood. ( b – f ) Phyllosoma larval stage of palinurid decapod crustaceans. ( b ) General view showing symmetrical network of diverticula branching off from midgut. ( c ) Blind-ended diverticula. ( d ) Bifurcating diverticula (red arrows). ( e ) Diverticula filled with fluid food. ( f ) Histological section through diverticulum (note large vacuoles in digestive cells). ( g ) Section through the hepatopancreas of Nephrops norvegicus (Decapoda) showing typical closely packed digestive tubules. ( h , i ) Speleonectes atlantida [40] (remiped crustacean) from submarine cave, Canary Islands, showing orange-coloured midgut with numerous lateral pairs of outpocketings (yellow arrows indicate segment boundaries). di, diverticula; e, eye; fg, foregut; he, head; hs, head shield; lu, lumen; m, mouth; mg, midgut; mgo, midgut outpocketing; pd, primary duct; ta, trunk appendage; ts, trunk segment; va, vacuole. All light micrographs. a , courtesy A. Avenant-Oldewage; e , f , S. Mikami; g , D.M. Neil; h , i , U. Streker, http://www.naturalanza.com . Scale bar, 5 mm for b , h , i ; 1 mm for a , c ; 500 μm for d , 100 μm for e , f ; and 25 μm for g . Full size image Megadictyon , Jianshanopodia and Pambdelurion are remarkable for their well-developed digestive glands and also for their large size, with lengths exceeding 10 times that of other coeval lobopodians with cylindrical undifferentiated alimentary tracts [5] , [17] , [20] , [42] , [43] , [44] . Also remarkable are their probably prehensile frontal appendages, funnel-like pharynx lined with cuticular teeth recalling that of Recent and Cambrian priapulid worms [45] , [46] , [47] and teeth complex encircling the mouth opening [48] ( Fig. 4 and Supplementary Fig. 2 ). When considered together with the digestive glands described here, these features suggest the ability to manipulate food via macrophagous habits and to digest it via enzymatic breakdown. These animals are interpreted here as some of the earliest potential macropredators. Possible arthropod remains within the gut of Pambdelurion ( Supplementary Fig. 4l ) support this interpretation, although scavenging cannot be excluded. The stout, conical lobopods of Megadictyon and Jianshanopodia suggest an epibenthic lifestyle whereas the flap-like lobes of Pambdelurion may indicate some swimming abilities. 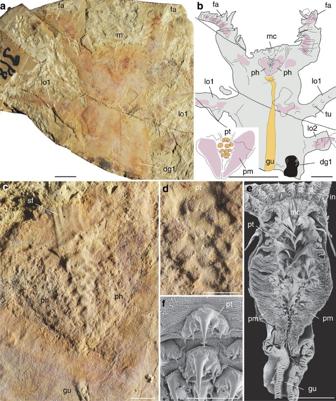Figure 4: Pharyngeal structure of the Early Cambrian lobopodianJianshanopodiawith analogues in Recent priapulid worms. (a–d)Jianshanopodia decora, ELI-J001, incomplete specimen, general views showing anterior part of body, close-up of mouth and pharynx region lined with teeth. (e,f)Priapulus caudatus(Recent, Sweden), longitudinal section through introvert showing thick pharyngeal muscle structure and pharyngeal teeth, and details of teeth arrangement.e,fare scanning electron micrographs. Body in grey, presumed muscle remains in pink, digestive gland in black, and pharyngeal teeth and gut in orange. dg1, first pair of digestive glands; fa, frontal appendage; gu, gut; in, introvert; lo1, 2, first and second pair of lobopods; m, mouth; mc, mouth cone; ph, pharynx; pm, presumed pharyngeal muscles; pt, pharyngeal tooth; sf, assumed sclerotized, circum-oral features; tu, tubercle. Scale bar, 10 mm fora,b; 2 mm forc–e; and 500 μm forf. Figure 4: Pharyngeal structure of the Early Cambrian lobopodian Jianshanopodia with analogues in Recent priapulid worms. ( a – d ) Jianshanopodia decora , ELI-J001, incomplete specimen, general views showing anterior part of body, close-up of mouth and pharynx region lined with teeth. ( e , f ) Priapulus caudatus (Recent, Sweden), longitudinal section through introvert showing thick pharyngeal muscle structure and pharyngeal teeth, and details of teeth arrangement. e , f are scanning electron micrographs. Body in grey, presumed muscle remains in pink, digestive gland in black, and pharyngeal teeth and gut in orange. dg1, first pair of digestive glands; fa, frontal appendage; gu, gut; in, introvert; lo1, 2, first and second pair of lobopods; m, mouth; mc, mouth cone; ph, pharynx; pm, presumed pharyngeal muscles; pt, pharyngeal tooth; sf, assumed sclerotized, circum-oral features; tu, tubercle. Scale bar, 10 mm for a , b ; 2 mm for c – e ; and 500 μm for f . Full size image Numerous Cambrian arthropods from exceptional biotas have well-preserved digestive systems with biserial midgut glands that display a variety of shapes from simple, short, bunch-like or lobe-like diverticula to extensive branching features (for example, naraoiids [49] ). They have been interpreted as digestive glands [49] , [50] in stem lineage arthropods such as Kerygmachela [22] , [51] ( Supplementary Fig. 3 ), Opabinia [52] , [53] ( Fig. 5a–c ) and Anomalocaris [26] , [54] ( Fig. 5f,g ), as well as in the early crown group arthropod Naraoia [47] ( Fig. 6f ). Phosphatized digestive glands have been described in several Cambrian arthropods, including Isoxys [7] , [55] ( Fig. 5d,e ), Leanchoilia [49] ( Fig. 5h–j ), Sidneyia [56] and various trilobites [57] . This type of gland preservation has almost exclusively been observed in fossil arthropods, which suggests that these animals, like their modern representatives, probably stored calcium and phosphate ions within their digestive tissues [57] . Optimal conditions during early mineralization before degradational collapse may have led to the preservation of microscopic internal features (100–120-μm-thick planar elements and 2–3 μm microspheres in Leanchoilia [47] ), whereas the featureless phosphatic digestive glands of Opabinia ( Fig. 5a–c ) probably resulted from preservation under less favourable conditions. The digestive glands of these arthropods are likely the same type as those of the large lobopodians, as shown by their phosphatic preservation, radiating internal microstructures, abaxial position, connection to the midgut and metameric arrangement. 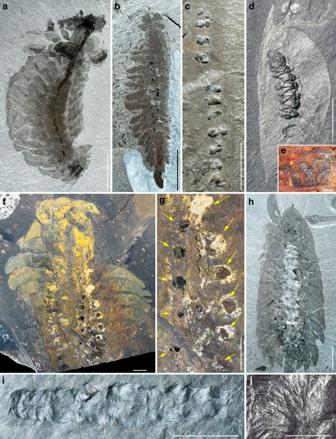Figure 5: Digestive glands in other arthropods from the Middle Cambrian Burgess Shale. (a–c)Opabinia regaliswith 11 pairs of digestive glands. (a) ROM 59873, general view. (b) ROM 59872, general view. (c) ROM 59874, details of digestive glands. (d)Isoxys acutangulus, ROM 57912 with possibly 11 pairs of digestive glands preserved in three dimensions. (e)Isoxyssp.54from the Early Cambrian Maotianshan Shale, China, CFM 00047 showing the tubular structure of digestive glands. (f,g) Anomalocaris canadensis,GSC 75535, general view and details of possibly six pairs of digestive glands (yellow arrows). (h–j)Leanchoilia superlata, ROM 54215, general view and details of closely packed digestive glands with ramified diverticula. Scale bar, 10 mm fora–c,f,g; 5 mm ford,h,i; 1 mm forj; and 500 μm fore. Figure 5: Digestive glands in other arthropods from the Middle Cambrian Burgess Shale. ( a – c ) Opabinia regalis with 11 pairs of digestive glands. ( a ) ROM 59873, general view. ( b ) ROM 59872, general view. ( c ) ROM 59874, details of digestive glands. ( d ) Isoxys acutangulus , ROM 57912 with possibly 11 pairs of digestive glands preserved in three dimensions. ( e ) Isoxys sp. [54] from the Early Cambrian Maotianshan Shale, China, CFM 00047 showing the tubular structure of digestive glands. ( f , g ) Anomalocaris canadensis, GSC 75535, general view and details of possibly six pairs of digestive glands (yellow arrows). ( h – j ) Leanchoilia superlata , ROM 54215, general view and details of closely packed digestive glands with ramified diverticula. Scale bar, 10 mm for a – c , f , g ; 5 mm for d , h , i ; 1 mm for j ; and 500 μm for e . 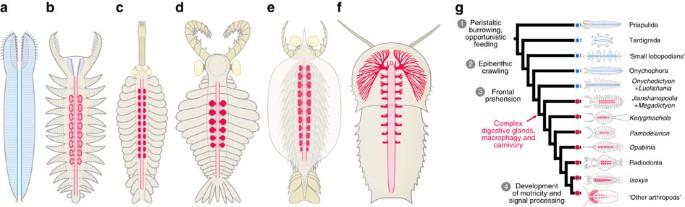Figure 6: Digestive systems and arthropod evolution. (a) Priapulid worm with a straight gut lacking digestive glands. (b–f) Panarthropods with complex paired digestive glands exemplified byJianshanopodia,Opabinia,Anomalocaris,IsoxysandNaraoia. All simplified dorsal views emphasizing the digestive system. (g) Simplified cladogram based on recent cladistic studies1,2,3,4,6,7,51. Blue dots indicate lineages in which digestive glands are lacking, red dots indicate lineages that have sophisticated digestive systems. Other innovations in the evolutionary history of arthropods are indicated alongside the cladogram. 1, Unsegmented worms such as priapulids used peristaltic contractions for locomotion; 2, paired locomotory appendages allowed crawling and climbing (for example, lobopodians); 3, frontal appendages with prehensile function facilitated feeding; and 4, more complex brains11,12and optic lobes enhanced motor and sensory abilities. ‘Small lobopodians’ refer to lobopodians with non-articulated trunk appendages and no specialized head appendages such asPaucipodia, Microdictyon, CardiodictyonandHallucigenia. ‘Radiodonta’ are animals with multi-articulated frontal appendages and complex mouth apparatus with teeth-like sclerotized elements, typically anomalocaridids. ‘Other arthropods’ encompass more advanced stem and crown group arthropods. Full size image Figure 6: Digestive systems and arthropod evolution. ( a ) Priapulid worm with a straight gut lacking digestive glands. ( b – f ) Panarthropods with complex paired digestive glands exemplified by Jianshanopodia , Opabinia , Anomalocaris , Isoxys and Naraoia . All simplified dorsal views emphasizing the digestive system. ( g ) Simplified cladogram based on recent cladistic studies [1] , [2] , [3] , [4] , [6] , [7] , [51] . Blue dots indicate lineages in which digestive glands are lacking, red dots indicate lineages that have sophisticated digestive systems. Other innovations in the evolutionary history of arthropods are indicated alongside the cladogram. 1, Unsegmented worms such as priapulids used peristaltic contractions for locomotion; 2, paired locomotory appendages allowed crawling and climbing (for example, lobopodians); 3, frontal appendages with prehensile function facilitated feeding; and 4, more complex brains [11] , [12] and optic lobes enhanced motor and sensory abilities. ‘Small lobopodians’ refer to lobopodians with non-articulated trunk appendages and no specialized head appendages such as Paucipodia, Microdictyon, Cardiodictyon and Hallucigenia . ‘Radiodonta’ are animals with multi-articulated frontal appendages and complex mouth apparatus with teeth-like sclerotized elements, typically anomalocaridids. ‘Other arthropods’ encompass more advanced stem and crown group arthropods. Full size image Most recent phylogenies of Ecdysozoa based on molecular and morphological data [1] , [2] , [3] , [4] , [5] , [6] , [7] , [8] , [51] place priapulid worms within the Cycloneuralia [58] , a sister group of Panarthropoda (Arthropoda, Tardigrada, Onychophora), and suggest a divergence time preceding the rise of panarthropods [3] . No Cambrian priapulid [45] , [47] has a complex digestive system. Instead, they possess a straight cylindrical gut connecting their teeth-bearing muscular pharynx to the anus [46] . By analogy to their modern representatives [46] , extracellular digestion via enzymes secreted along the gut epithelium is the most obvious process by which Cambrian priapulids digested and assimilated food. Among the basal panarthropods is a great variety of small lobopodians ( Fig. 6 ) exemplified by Paucipodia, Hallucigenia, Cardiodictyon, Microdictyon, Onychodictyon, Luolishania , Miraluolishania and Diania , all possessing tubular guts without diverticula. The digestive glands exhibited by large lobopodians seem to represent an important anatomical novelty with major implications for the evolution of arthropods ( Fig. 6 ). By contrast with simple tubular guts, these features increase the surface exchange between nutrients and epithelial tissues where enzymatic breakdown and assimilation takes place. They would have created a more efficient way to transform food into energy with at least two possible implications. First, digestive glands allowed arthropods to digest larger food particles (macrophagy). This might have been all the more important considering that most Cambrian arthropods did not possess the array of highly differentiated (for example, cephalic) appendages that allow modern arthropods to process food before ingestion and digestion. Second, digestive glands allowed arthropods to obtain more energy with greater efficiency such that they could exploit a more diverse array of food sources. As animals themselves evolved and radiated, they created a food source (live prey and carcasses) that required enzymatic breakdown of complex molecules such as proteins and lipids. Acquiring the capability to extract energy from nutrient-rich animal matter more efficiently using specialized digestive organs may have given arthropods the considerable advantage of being able to maintain higher energy demands. Arthropods are among the most mobile animals in the Cambrian ecosystem with a variety of crawlers, swimmers and hunters [13] , [26] , [55] , [59] , implying high metabolic requirements. Digestive glands likely played a key role in promoting carnivory via predation and scavenging. Digestive organs of comparable adaptive value are likely to have developed independently in other metazoan lineages. Paired digestive glands are known in a variety of non-arthropod extant groups [21] such as annelids (for example, multicaecate gut of Aphrodita ; paired caeca of hirudinoid; branched diverticula in myzostomid polychaetes), turbellarians, molluscs (for example, nudibranch gastropods such as Embletonia ) and nemerteans (gastrovascular cavity with lateral branchings). However, fossil evidence for digestive glands in Cambrian non-arthropod groups is rare and uncertain (for example, the lophotrochozan Odontogriphus [60] ). It is also important to note that the lack of digestive glands does not necessarily preclude carnivory and macrophagy altogether, but their presence may have increased the speed and efficiency of chemical food processing and allowed for more active predation strategies. Recent priapulid worms and their Cambrian ancestors are predators without digestive glands [47] , but they typically have a less mobile, infaunal mode of life. We are not equating the presence of digestive glands with strict carnivory. Numerous Recent herbivorous/detrivorous or omnivorous crustaceans (for example, many atyiid shrimps [61] ) also have such glands. One should not exclude that some Cambrian arthropods had such diverse diets and opportunistic behaviours, in addition to predation. On the basis of current knowledge, arthropods are the Cambrian animal group in which sophisticated digestive systems became best developed. Combined with a suite of major innovations relating to motility and motricity (for example, more complex brains [11] , [12] , visual organs [59] , and feeding and locomotion (for example, appendage specialization [62] ), sophisticated digestive systems are likely to have been of major importance in the ecological success of arthropods. Their extensive diversification and disparate modes of life allowed them to maintain a pivotal role in the dynamics of benthic and pelagic ecosystems from the Cambrian up until today. Recent studies [63] based on modern ecological analogues have emphasized the role of oxygen (environmental trigger) in the spreading of carnivory (ecological driver) and how it might explain the expansion of animal diversity at the beginning of the Cambrian by escalation and coevolution [63] . Nonetheless, the ability to exploit diverse food sources via sophisticated digestive systems was likely a driving factor in the evolution of arthropods and the further elaboration into complex trophic webs. Analyses of fossils Specimens examined are listed in Supplementary Table 1 , and are housed in the Early Life Institute in Xi’An, China; the Museum Geologicum Universitatis Hauniensis in Copenhagen, Denmark; the Royal Ontario Museum in Toronto, Canada; and the Canadian Geological Survey in Ottawa, Canada. Fossils were photographed with a D3X Nikon camera, an EOS 500D Canon camera, a Leica MZ125 stereomicroscope and a FEI Quanta 250 field emission scanning electron microscope at 15 kV in low and high vacuum using secondary and backscattered electron detectors. SEM-EDS was performed with SAMx EDX-SDD spectrometer. Figures were prepared with Adobe Photoshop CS5 and Adobe Illustrator CS4. How to cite this article: Vannier, J. et al. Sophisticated digestive systems in early arthropods. Nat. Commun. 5:3641 doi: 10.1038/ncomms4641 (2014).